Strain response of thermal barrier coatings captured under extreme engine environments through synchrotron X-ray diffraction The mechanical behaviour of thermal barrier coatings in operation holds the key to understanding durability of jet engine turbine blades. Here we report the results from experiments that monitor strains in the layers of a coating subjected to thermal gradients and mechanical loads representing extreme engine environments. Hollow cylindrical specimens, with electron beam physical vapour deposited coatings, were tested with internal cooling and external heating under various controlled conditions. High-energy synchrotron X-ray measurements captured the in situ strain response through the depth of each layer, revealing the link between these conditions and the evolution of local strains. Results of this study demonstrate that variations in these conditions create corresponding trends in depth-resolved strains with the largest effects displayed at or near the interface with the bond coat. With larger temperature drops across the coating, significant strain gradients are seen, which can contribute to failure modes occurring within the layer adjacent to the interface. Thermal barrier coatings (TBCs) have played a significant role in advancing the efficiency of turbine engines over the years. These high-temperature ceramic coatings provide a high level of thermal protection for the underlying turbine substrate while exhibiting durability under extreme environmental conditions [1] , [2] , [3] . While their effect on the jet engine efficiency has solidified the use of TBCs in industry during the past decades, research to extend the life and performance of TBCs is still needed. Further understanding of the complex mechanics related with these multi-layered coatings is required to link different thermal and mechanical operating conditions with common failure mechanisms such as delamination and spallation. Owing to mismatch of the thermal expansion of different layers along with extreme temperature changes between coating manufacturing, operating temperatures and shutdown periods, large residual stresses are present in each of the layers of the coating. This is especially true for the thermally grown oxide (TGO) layer, which develops at the bond coat/TBC interface and is known to exhibit compressive residual stresses >1 GPa (refs 4 , 5 , 6 , 7 ). Therefore, strains in this region are critical to understanding the link between thermal and mechanical operating conditions and various failure modes of the coatings. Many studies have shown that damage initiation for some failure modes occurs at this bond coat/TGO/TBC interface [2] , [3] , [4] , [7] , [8] , [9] , [10] , [11] , [12] , [13] , [14] , [15] , [16] , [17] , [18] , [19] , [20] , [21] , [22] , [23] . The strain behaviour of the layers at high temperature is largely related to the thermal gradient across the coating due to internal cooling of the turbine blade and mechanical loads from centrifugal forces in combination with the temperature-dependent thermal and mechanical properties of the coating. In the presence of sufficient thermal gradients, crack initiation and propagation have been seen to develop in the TBC parallel to the interface [24] , [25] . It has also been shown that with reduced applied mechanical loads, failure modes in the bond coat are suppressed, which shifts failure modes towards delamination of the TBC [26] . Combinations of both thermal gradients and mechanical loads have been applied through novel cylindrical sample geometries to establish that thermal gradient mechanical fatigue loading results in the development of cracks beneath the top coat and further the spallation process [27] . While research in the fatigue studies of TBC coatings is abundant, these efforts have generally been ex situ investigations of failure propagation after cycling. Significant strides in understanding the causes of different failure modes can be made by the acquisition of high-temperature in situ data through novel measurement techniques. New experimental techniques are being developed in which these strains can be measured in situ with variation of loading conditions at high temperatures [28] , [29] . With the use of high-energy synchrotron X-rays, through sample transmission can be used to measure high spatial and strain resolution through the thickness of internal layers of the coating [30] . Synchrotron X-ray diffraction (XRD) has been used to show how depth-resolved phases and residual stresses evolve after thermally ageing plasma-sprayed TBCs [31] . With the speed at which measurements are taken, high-energy XRD can provide the ability to accurately capture transient material behaviour such as creep and plasticity. This method has previously been used to quantify residual stresses in the various layers under high-temperature conditions [25] , [32] . More recently, synchrotron XRD strain measurements on TBCs under uniform thermal loading have shown the dependence on applied axial loads of the strain transition into the tensile region at high temperature in the TGO of as-coated specimens [29] . The work presented here uses high-energy synchrotron X-rays to measure in situ internal strains as a thermal gradient and mechanical load are applied to the coating. This is done so with a tubular specimen and X-ray beam orientation shown in Fig. 1a . The novel experiment developed, produced valuable information on depth-resolved strains as both thermal gradient and mechanical loading are varied at elevated temperatures. Displayed here are previously unseen relationships between internal strains and operating conditions directly determined from experimental measurement. 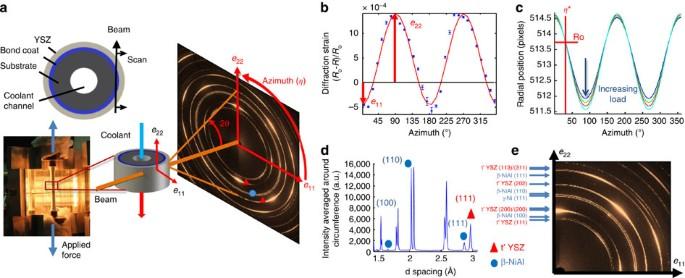Figure 1: Experimental set-up for loading and synchrotron measurements. (a) Thermal gradient loading of cylindrical samples maintaining access for synchrotron XRD measurement transmitting through the sample tangential to the layers yielding 2D diffraction with radial (e11) and axial (e22) strains, (b) 2D strain measured from radial deviation around the azimuth of (110) diffraction ring, (c) determination of (100) strain-free azimuth reference angle (η*) and strain-free radius (Ro) using variable mechanical load, (d) phase identification displaying intensity averaged around circumference of diffraction ring versus d-spacing, (e) raw data highlighting lattice planes of phases. Figure 1: Experimental set-up for loading and synchrotron measurements. ( a ) Thermal gradient loading of cylindrical samples maintaining access for synchrotron XRD measurement transmitting through the sample tangential to the layers yielding 2D diffraction with radial ( e 11 ) and axial ( e 22 ) strains, ( b ) 2D strain measured from radial deviation around the azimuth of (110) diffraction ring, ( c ) determination of (100) strain-free azimuth reference angle ( η *) and strain-free radius ( R o ) using variable mechanical load, ( d ) phase identification displaying intensity averaged around circumference of diffraction ring versus d-spacing, ( e ) raw data highlighting lattice planes of phases. Full size image This study used as-coated tubular IN100 specimens, with inner and outer radii of 2 and 4 mm, which allowed for the heating of the outer coated surface and cooling of the inner substrate surface to create a thermal gradient across the coating layers. The electron beam physical vapour deposition (EB-PVD) early-cycled TBC system on the sample consisted of 7–8 wt% yttria-stabilized zirconia (YSZ) ceramic top coat with a thickness of 211±4 μm, a TGO thickness of ~0.3 μm, and a NiCoCrAlY bond coat with a thickness of 118±4 μm. It should be noted that the same sample was used throughout the experiments where roughly three 80-min cycles were completed before the presented cycles. To investigate the strain behaviour under loading conditions relevant for gas turbine blades in aircraft engines, three types of experiments were conducted: (i) single flight cycles, (ii) mechanical tests at various temperatures up to 1,000 °C and (iii) thermal gradient tests at high temperature. For single flight cycle tests (i), the outer surface temperature was ramped up through duration of 20 min to 1,000 °C and held for 40 min before ramping down to room temperature while maintaining a constant mass flow of cooling air and a mechanical load resulting in 64 MPa nominal stress. The strain response to mechanical loading (ii) was tested through repeated stepwise mechanical load increases at five different homogeneous temperatures (no superposed thermal gradient) from room temperature up to 1,000 °C. To isolate the strain effects from thermal gradient (iii), the sample was uniformly heated to a high temperature of 1,000 °C. The inner surface of the substrate was then cooled slowly while the surface temperature was held constant. These novel measurements have revealed previously unseen in situ strain response of the TBC that can contribute towards enhancing coating lifespans. Diffraction peaks The results for these experiments were analysed for multiple phases as shown in Fig. 1d . The phases are identified in the X-ray spectrum with the beam penetrating directly through the bond coat, giving phases for both bond coat and YSZ due to the curvature of the sample. In the YSZ, the t′-YSZ is the most prominent phase measured. Two prominent phases are detected in the bond coat. These are the β-NiAl phase and a solid solution γ-Ni phase. Strain results will be shown for the bond coat β-NiAl phase and the t′-YSZ phase. Displayed in Fig. 1e is a raw data image highlighting the lattice planes of these phases. Due to the EB-PVD application process, the YSZ top coat consists of a columnar structure normal to the bond coat surface. This results in texturing with a preferred orientation displayed in Fig. 2 . This displays the measured intensity versus ring azimuth angle from 0 to 360° for YSZ (111), YSZ (200) and NiAl (110). The texturing displayed here for the YSZ is measured with an X-ray beam tangential to the cylindrical surface, providing a two-dimensional (2D) measurement plane that is parallel to the YSZ columns. In comparison, the NiCoCrAlY bond coat exhibits randomly oriented grains. The texturing of similarly manufactured samples can also be seen in other work [33] . The TGO layer, which is expected to be α-Al 2 O 3 , was not detectable in the diffraction data that is attributed to its minimal thickness in these early-cycled specimens. Future work will include studies of pre-cycled specimens from which the TGO signal, including strain state, is expected to be measurable. 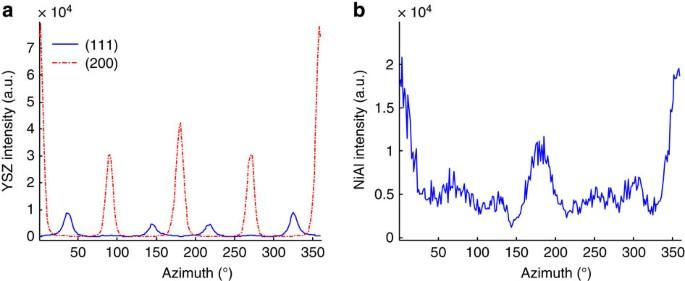Figure 2: Display of texturing through azimuthally dependent intensity. Texturing displayed through intensity versus azimuth for (a) YSZ (111) and (200), and (b) NiAl (110). Figure 2: Display of texturing through azimuthally dependent intensity. Texturing displayed through intensity versus azimuth for ( a ) YSZ (111) and (200), and ( b ) NiAl (110). Full size image Single flight cycle strain evolution For the single flight cycle measurement, the outer surface is exposed to a temperature profile with ramp-up and then held at high temperature while the internal cooling and applied mechanical load are held constant. The cycle shown in Fig. 3 was conducted at 75 standard litres per minute (75%) and 64 MPa nominal tensile stress. The strain of a single location is shown for both the bond coat and YSZ throughout a single flight cycle. These locations are near the bond coat/top coat interface as shown. The strain results for NiAl for a single location throughout the cycle are shown in Fig. 3d and include lattice planes of both (100) and (110). Throughout temperature increase from room temperature to 1,000 °C, the strain ratio of the (100) to (110) planes varies between 1.6 and 2.2. This highlights the anisotropy of the NiAl phase. It also validates the strain values as the elastic modulus ratio of the two planes is very close to the inverse of the strain ratio. Room temperature elastic moduli for the (100) and (110) were calculated to be 97 and 188 GPa, respectively, from experimentally determined elastic compliance constants [34] . Owing to the fine-grained nature of the bond coat, anisotropy is only seen in the scale of micro-strain. 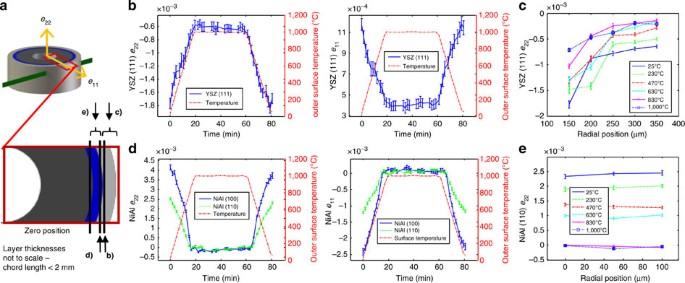Figure 3: Strain measurements for a single cycle. Loading conditions of 64 MPa nominal mechanical stress and cooling air mass flow of 75 standard litres per minute were applied to the specimens. (a) Through transmission measurement locations relative to the coating cross-section displaying single locations at the interface as well as through layer scans, (b) YSZ (111) axial (e22) and radial (e11) strains, (c) YSZ (111)e22strain through depth during thermal ramp-up, (d) bond coat NiAl (100) and (110) axial (e22) and radial (e11) strains, (e) bond coat NiAl (110)e22strain through depth during thermal ramp-up. Figure 3: Strain measurements for a single cycle. Loading conditions of 64 MPa nominal mechanical stress and cooling air mass flow of 75 standard litres per minute were applied to the specimens. ( a ) Through transmission measurement locations relative to the coating cross-section displaying single locations at the interface as well as through layer scans, ( b ) YSZ (111) axial ( e 22 ) and radial ( e 11 ) strains, ( c ) YSZ (111) e 22 strain through depth during thermal ramp-up, ( d ) bond coat NiAl (100) and (110) axial ( e 22 ) and radial ( e 11 ) strains, ( e ) bond coat NiAl (110) e 22 strain through depth during thermal ramp-up. Full size image At room temperature, the bond coat shows a very large tensile residual strain in the in-plane ( e 22 ) direction. As it is ramped up to high temperature, it then relaxes to zero strain. The bond coat NiAl has displayed a changing e 22 strain per temperature rate for above and below 600 °C. The (100) plane strain rate was −3.95E−6 (mm per mm) per °C between 25 and 600 °C while increasing in magnitude to −4.95E−6 (mm per mm) per °C, between 600 and 1,000 °C. A ductile to brittle transition, associated with the activation of grain boundary creep, has been reported in literature at similar temperatures around 600 °C (ref. 35 ) for the bond coat and is likely to have an influence here. As can be seen by the strain slope above 600 °C, the strain linearly relaxes to zero strain at 800 °C. At this point, no further changes in strain can be seen with increased temperature. The shift to near zero strain at high temperature is expected due to the TBC’s manufacturing temperature of 1,000 °C. During temperature shifts from application and operating temperatures to room temperature, the TBC system develops large residual stresses as the layers contract at different rates. Figure 3b displays the YSZ (111) strain near the interface throughout a cycle. The YSZ exhibits compressive in-plane ( e 22 ) strains at room temperature displaying that the YSZ exhibits a smaller thermal expansion coefficient relative to the bond coat and substrate. It also displays a similar shift to near zero at high temperature with some remaining compressive e 22 residual strain. The through-thickness plot shows that the largest shift during temperature ramp-up along with the largest high-temperature residual strains occur at the interface. This observation can be attributed to the specific microstructure of EB-PVD YSZ coatings that display a gradient in porosity, corresponding to a gradient in elastic modulus, from low porosity near the interface to increasing porosity towards the surface. These in-cycle results highlight the importance of strains near the interface during cyclic conditions. Strain gradients across the layers provide valuable information on the loading state as well as the material’s behaviour. Strain response to mechanical loading at temperature The effects of mechanical loading at various temperatures are shown in Fig. 4 . Locations in both the bond coat and YSZ, near the interface, were monitored as the applied load ramped up with nominal stresses of 16, 32, 48 and 64 MPa at each temperature. Displayed in Fig. 4c,d are the changes in e 22 strain versus changes in applied nominal stresses for bond coat and YSZ, respectively. This displays that the NiAl in the bond coat gradually bears less of the applied load as temperature increases. This is demonstrated by the decreasing slope of the strain to applied stress with increasing temperatures. At 800 and 1,000 °C, the slope of strain of the bond coat to nominally applied load, is near zero and also exhibits zero strain shift between temperatures. As the micro-strains averaged over the grains only displays elastic strain, this highlights the existence of inelastic behaviour (plasticity and creep) in the bond coat at and above 800 °C. The same trend occurs in the YSZ layer. As the temperature moves towards operating temperatures, it converges to zero load bearing. The lack of micro-strain present internally within the NiAl grains at elevated temperature with increased loads suggests the possibility of sliding of the grain boundaries between the NiAl and Ni phases that could affect the structural integrity of the bond coat over cycling. 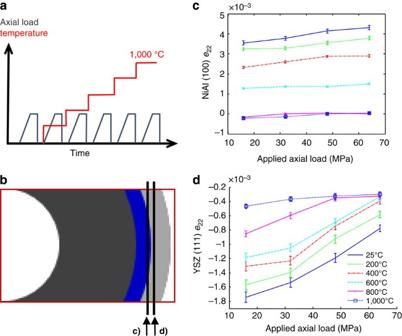Figure 4: Strain effects due to variations in mechanical load. (a) Loading conditions displaying mechanical load cycles conducted at each homogeneous temperature, (b) measurement locations near the interface for both the bond coat and YSZ, (c) NiAl (111)e22strain versus applied mechanical load at various temperatures, (d) YSZ (111)e22strain versus applied mechanical load at various temperatures. Figure 4: Strain effects due to variations in mechanical load. ( a ) Loading conditions displaying mechanical load cycles conducted at each homogeneous temperature, ( b ) measurement locations near the interface for both the bond coat and YSZ, ( c ) NiAl (111) e 22 strain versus applied mechanical load at various temperatures, ( d ) YSZ (111) e 22 strain versus applied mechanical load at various temperatures. Full size image Strain effects from thermal gradients Variation of thermal gradient at high temperature was studied for its strain effects in the bond coat and YSZ. 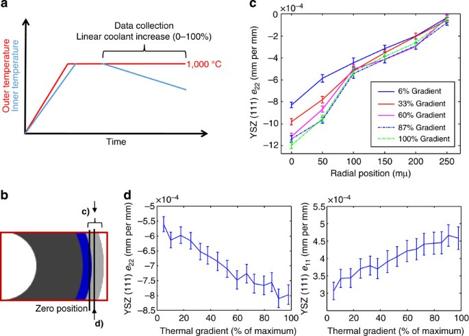Figure 5: Strain effects due to variations in thermal gradient. (a) Thermal loading of the sample with linear increase in the imposed thermal gradient, (b) YSZ measurement locations displayed at single location adjacent to interface as well as a scan through thickness, (c) YSZ (111)e22strain displayed through the YSZ thickness at various thermal gradients, (d) YSZ (111)e22ande11strains at ~75 μm distance from the interface versus thermal gradient. Figure 5 displays the e 22 strain results as the thermal gradient was increased from 0 to 100% of maximum thermal gradient, corresponding to an approximate maximum temperature drop across the YSZ layer of 150 °C per 211 μm. This rough estimate of thermal gradient was approximated using the change in d-spacing across the layer along with the measured relationship between applied temperature and d-spacing. At high temperature, the bond coat displayed no variation in strain due to thermal gradient. However, the gradient has an effect on the YSZ strains, which is substantial near the interface with the bond coat. Figure 5c shows that with increasing thermal gradient, the YSZ demonstrates minimal change in strain from the outer surface into the middle of the layer, whereas the inner region of the YSZ displays a significantly increasing compressive strain and thus higher strain gradient. Figure 5: Strain effects due to variations in thermal gradient. ( a ) Thermal loading of the sample with linear increase in the imposed thermal gradient, ( b ) YSZ measurement locations displayed at single location adjacent to interface as well as a scan through thickness, ( c ) YSZ (111) e 22 strain displayed through the YSZ thickness at various thermal gradients, ( d ) YSZ (111) e 22 and e 11 strains at ~75 μm distance from the interface versus thermal gradient. Full size image The observed strain response on the variation of thermal gradient by means of variation of cooling air mass flow can be attributed to a combination of several effects, related to the microstructure and the specimen geometry. The EB-PVD coating has a higher density at and near the interface than towards the surface with a high gradient in porosity near the interface up to about 100 μm distance to the interface. With increasing distance from the interface the porosity does not change much. Consequently, the thermal conductivity and the elastic modulus of the coating decrease with distance from the interface, resulting in opposite effects on the strain. The effect of an increase in thermal conductivity is a decrease of a thermal gradient in the case of a constant heat flux. A decrease in thermal gradient would result in a decrease of strain gradient if the elastic properties were homogeneous. Since in the case of columnar EB-PVD YSZ coatings the macroscale elastic modulus displays a gradient that increases towards the interface, strain and strain gradients in the YSZ phase would increase towards the interface if the thermal gradient would be constant. The tubular specimen geometry results in an increase of heat flux from the outer surface to the cooled inner surface that would result in an increasing thermal gradient towards the interface if the thermal conductivity would be homogeneous. In addition to the microstructural effects, the reduction in temperature near the interface can also reduce the level of unmeasured inelastic strain present. A combination of the listed effects could create or contribute to the trends in changing strain gradient across the thickness as is displayed here. Combining the results from the different experiments, the findings from this study will contribute to making significant steps towards extending the life span of TBCs by providing previously unknown material behaviour under extreme environments. This will be used to validate models and close the design loop in creating more durable coatings by adjusting the processing parameters as well as through more innovation in enhancing coating materials. Having knowledge of how internal strains react to different operating conditions, including the applied thermal gradient, increases our ability to define the focus of TBC research to reduce damage propagation in regions of the turbine blade that lead to early failure. These results have displayed a relation between increases in thermal gradient and increase in stress gradient in the YSZ inner region, strengthening the assumption that a link can be made between thermal gradient and failure modes in the YSZ [24] . Results also emphasize the importance of mechanical load in regions of the turbine blade and its link to damage propagation in the bond coat due to the presence of plastic strain. Future experiments will show how these dependencies on operating conditions vary throughout the life span of a turbine blade. Continuing studies using these new measurement techniques can lead to significant advances in performance and durability of these coatings. In situ thermal gradient mechanical set-up To heat the sample, a heater containing four 2,000 W lamps with elliptical mirrors encircling the specimen was used to focus the energy as shown in Fig. 1 . YSZ surface temperatures were controlled up to 1,000 °C while the thermal drop across the coating was controlled by the mass flow of pressurized air having ambient temperature through the centre of the sample. Mass flow could be controlled between 0 and 100 standard litres per minute. Tensile nominal mechanical stresses of 16–128 MPa were applied to simulate the centrifugal loads on turbine blades. To maintain access for beam diffraction, circular inlet and exit windows were created through the centre of the front and back of the heater wall. Further information on the experimental set-up can be found in the previous work [28] . Measurement methods Throughout all experiments, the beam scanned through the coating layers with a window and step size of 50 μm. This gives depth-resolved strain measurements during transient loading conditions. With high-energy synchrotron X-rays and a 2D detector, diffraction measurements in 360° are projected onto the detector plane perpendicular to the through transmission beam as shown in Fig. 1 . Measurements were taken with a beam energy of 65 keV, resulting in full-diffraction rings to a d-spacing as low as 1.29 Å. High-resolution strain measurements were taken with a 200-μm pixel size 2D detector at a distance of 1,500 mm that provides the radial deviation of the diffraction ring around the entire azimuth angle. Due to the geometry of grazing the coating layers tangentially, as shown in Fig. 1 , the beam chord length never exceeds 2 mm, reducing the time required to achieve quality images down to five frames of 1-s exposure time each for a window size of 50 × 300 μm (width by height). Synchrotron diffraction strain analysis Diffraction rings are recorded for each lattice plane in the multiple coating layers using an 85-s scan with 10 discretized steps through the coating thickness. As the lattice structure is strained in the directions shown, the patterns are measured as elliptical rings. These micro-strains measured within the grains provide the elastic strain response of each phase. This elliptical deviation from a circle with a strain-free radius provides the deviatoric micro-strain tensor for that lattice plane [36] . To measure the directional strain within the measurement plane, radial measurements of an individual ring are conducted around the azimuth angle, and compared with this strain-free radius, R o , as described by Diaz et al. [29] and shown in Fig. 1b . Strain-free radius values are determined from a method of measuring a strain-free azimuth angle, which is shown as η * in Fig. 1c . This method is further described in the work by Almer et al. [37] The reference angle, η *, is determined by measuring the distortion of the diffraction ring while applied tensile loading is increased. This provides the reference angle of which zero deviatoric strain occurs. This gives a value of R o at each measurement independent of temperature. The strain tensor calculations are then conducted using the fundamental strain equation [38] . The use of high-energy X-rays (65 keV) results in small Bragg angles, with 2 θ values for the peaks analysed between 2° and 6°. This means that the measured diffraction vectors are nearly aligned with the e 22 – e 11 plane, such that the coefficients in the fundamental strain equation for e 11 and e 22 are near unity while the e 33 coefficient is nearly negligible, with a value between 0.001 and 0.003. These radial ( e 11 ) and axial ( e 22 ) strains are averaged over distances from the interface due to the curvature of the coating. With the radial position being much greater than the coating thickness, the contribution of the circumferential strain component on the measured e 11 strain is expected to be minimal. Methods are being developed to convert strain to stress using X-ray elastic constants and various assumed stress states in the layers, as well as exploiting the anisotropic nature of the lattice strains within the grains to improve the approximation of the unknown stress direction parallel to the beam. How to cite this article: Knipe, K. et al. Strain response of thermal barrier coatings captured under extreme engine environments through synchrotron X-ray diffraction. Nat. Commun. 5:4559 doi: 10.1038/ncomms5559 (2014).